Thickness sorting of two-dimensional transition metal dichalcogenides via copolymer-assisted density gradient ultracentrifugation Two-dimensional transition metal dichalcogenides have emerged as leading successors to graphene due to their diverse properties, which depend sensitively on sample thickness. Although solution-based exfoliation methods hold promise for scalable production of these materials, existing techniques introduce irreversible structural defects and/or lack sufficient control over the sample thickness. In contrast, previous work on carbon nanotubes and graphene has shown that isopycnic density gradient ultracentrifugation can produce structurally and electronically monodisperse nanomaterial populations. However, this approach cannot be directly applied to transition metal dichalcogenides due to their high intrinsic buoyant densities when encapsulated with ionic small molecule surfactants. Here, we overcome this limitation and thus demonstrate thickness sorting of pristine molybdenum disulfide (MoS 2 ) by employing a block copolymer dispersant composed of a central hydrophobic unit flanked by hydrophilic chains that effectively reduces the overall buoyant density in aqueous solution. The resulting solution-processed monolayer MoS 2 samples exhibit strong photoluminescence without further chemical treatment. Molybdenum disulfide (MoS 2 ), one of the transition metal dichalcogenides (TMDs), has been studied with great interest for a wide range of applications due to its unique electronic, optical and catalytic properties [1] , [2] , [3] , [4] , [5] , [6] , [7] , [8] , [9] , [10] , [11] , [12] , [13] , [14] , [15] . The bulk MoS 2 crystal is a semiconductor with a 1.2 eV indirect bandgap and consists of covalently bonded S-Mo-S stoichiometric layers that interact with neighbouring layers via the relatively weak van der Waals interaction. When isolated as a single stoichiometric layer, MoS 2 shows strong visible photoluminescence due to the emergence of a 1.9 eV direct bandgap at the K point of the hexagonal Brillouin zone [2] , [8] , [16] . To fully understand and exploit the unique properties of single-layered MoS 2 , many production methods have been developed including micromechanical [1] , chemical [11] , [17] and surfactant-assisted liquid-phase exfoliation [18] , [19] , [20] , [21] , in addition to growth via chemical vapour deposition [22] . While the micromechanical cleavage technique produces single- or few-layered MoS 2 with high structural quality, this method lacks sufficient scalability for practical applications. On the other hand, solution-phase exfoliation of single-layered MoS 2 can be achieved by lithium intercalation, although this process drives a phase transition to the metallic 1T-MoS 2 structure, thus necessitating subsequent thermal treatments in an attempt to recover the semiconducting 2H-MoS 2 phase [11] , [23] . However, complete semiconducting phase recovery has not yet been demonstrated, and the presence of the residual metallic phase can have detrimental effects, especially in electronic applications. Alternative liquid exfoliation methods can avoid the metallic 1T-MoS 2 phase transition, but typically yield a range of MoS 2 flake thicknesses. Finally, ultrathin MoS 2 growth by chemical vapour deposition requires high temperature processing and subsequent transfer from the growth substrate, which is arguably more cumbersome than solution-based approaches. Here, we demonstrate an alternative solution-based route for preparing structurally pristine, ultrathin MoS 2 nanosheets via isopycnic density gradient ultracentrifugation (DGU). Originally used for biomolecule separations [24] , DGU has emerged as one of the leading techniques for isolating structurally and electronically monodisperse populations of carbon nanotubes [25] , [26] , [27] and graphene [28] . The physical structure of carbon nanomaterials coupled with their surrounding hydrated amphiphilic surfactants in aqueous solution leads to subtle buoyant density differences that drive separation to their respective isopycnic points when subjected to ultracentrifugation in a density gradient medium. In previous DGU studies on carbon nanomaterials, small molecule ionic surfactants, such as sodium cholate (SC), have proven to be exceptional dispersants that also enable exquisite control over the buoyant density as a function of the carbon nanomaterial physical and electronic structure [28] , [29] . Buoyant density model To assess the applicability of DGU to MoS 2 nanosheets, the following geometrical buoyant density model was used for SC-encapsulated MoS 2 : where ρ s =3.39 × 10 −7 g cm −2 is the sheet density of MoS 2 , N is the number of the MoS 2 sheets, m surf =7.15 × 10 −22 g is the mass of one SC molecule, σ =1.35 nm −2 is the surface packing density of SC on MoS 2 , ρ H2O is the density of water, t H =3.3 nm is the assumed hydration shell thickness, t MoS2 =0.67 nm is the MoS 2 interlayer distance, and t A =0.355 nm is the assumed anhydrous shell thickness. The values for σ , t H , and t A are based on previously established values for SC-encapsulated graphene [28] . The resulting buoyant densities are presented in Fig. 1c , where SC-encapsulated MoS 2 , even in the monolayer limit, is predicted to be more dense than iodixanol, the density gradient medium, at its solubility limit (1.32 g cm −3 ). Evidently, the relatively large sheet density of MoS 2 compared with graphene implies that the hydration of SC is insufficient to lower the buoyant density of suspended MoS 2 nanosheets to a level compatible with isopycnic DGU. 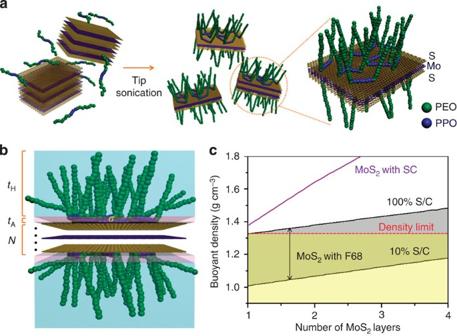Figure 1: Schematic illustration of the MoS2exfoliation process and buoyant density model. (a) Schematic of the MoS2exfoliation process in aqueous solution. In particular, MoS2flakes are exfoliated and dispersed by Pluronic F68 during tip ultrasonication. The brown and purple atoms are sulfur and molybdenum, and the green and blue spheres are PEO and PPO chains, respectively. (b) Buoyant density model for F68-encapsulated MoS2in aqueous solution, whereNis the number of MoS2layers,tAis the anhydrous layer thickness,tHis the hydration shell thickness, andσis the packing density. (c) Buoyant density model as a function of MoS2flake thickness. Black and purple lines represent scenarios where MoS2is encapsulated with F68 and sodium cholate (SC), respectively. The area enclosed by the two black lines indicates the possible buoyant density range that depends on the surface coverage of Pluronic F68 on MoS2. Isopycnic DGU separation of MoS2is only possible when the surfactant-encapsulated MoS2nanosheets have a buoyant density below the density limit imposed by the density gradient medium (red dashed line). Figure 1: Schematic illustration of the MoS 2 exfoliation process and buoyant density model. ( a ) Schematic of the MoS 2 exfoliation process in aqueous solution. In particular, MoS 2 flakes are exfoliated and dispersed by Pluronic F68 during tip ultrasonication. The brown and purple atoms are sulfur and molybdenum, and the green and blue spheres are PEO and PPO chains, respectively. ( b ) Buoyant density model for F68-encapsulated MoS 2 in aqueous solution, where N is the number of MoS 2 layers, t A is the anhydrous layer thickness, t H is the hydration shell thickness, and σ is the packing density. ( c ) Buoyant density model as a function of MoS 2 flake thickness. Black and purple lines represent scenarios where MoS 2 is encapsulated with F68 and sodium cholate (SC), respectively. The area enclosed by the two black lines indicates the possible buoyant density range that depends on the surface coverage of Pluronic F68 on MoS 2 . Isopycnic DGU separation of MoS 2 is only possible when the surfactant-encapsulated MoS 2 nanosheets have a buoyant density below the density limit imposed by the density gradient medium (red dashed line). Full size image To overcome this issue, we sought an alternative dispersant for MoS 2 that would enable greater hydration and thus lower buoyant density in aqueous solution. The nonionic, biocompatible, amphiphilic block copolymer Pluronic F68 was selected due to its relatively large molecular weight, long hydrophilic chains for effective steric hindrance, and its compatibility with the DGU process [30] . In particular, F68 is composed of a central hydrophobic polypropylene oxide (PPO) unit surrounded by hydrophilic polyethylene oxide chains ( Fig. 1a ), and is known to be effective as an amphiphilic dispersant for graphene [31] and DGU separation of carbon nanotubes [30] . To estimate the buoyant density of F68-encapsulated MoS 2 , the parameters in the aforementioned model are modified as following: m surf =1.40 × 10 −20 g is the mass of one F68 molecule, t A =1.6 nm, t H =20.6 nm and σ is varied between 0.058 and 0.575 nm −2 to account for the two likely extremes where the surface coverage of PPO chains on the MoS 2 surface ranges from 10–100%. While this model is oversimplified, it suggests that the buoyant density of F68-MoS 2 is substantially reduced compared with SC-MoS 2 and likely to fall within the achievable range of iodixanol-based density gradients, especially in the limit of ultrathin MoS 2 ( Fig. 1c ). Thickness sorting via density gradient ultracentrifugation To assess the effectiveness of F68-MoS 2 for DGU, 1 g of MoS 2 powder was first exfoliated and dispersed in 2% weight per volume (w v −1 ) aqueous solution of F68 via tip ultrasonication (See Supplementary Discussion for details). After ultrasonication, we found that 17.1% of the initial MoS 2 mass was dispersed, as determined by measuring the mass of the undispersed residual MoS 2 slurry. The resulting F68-MoS 2 dispersion was placed in a step density gradient and ultracentrifuged at 32 kr.p.m. for 24 h to remove thick MoS 2 flakes and enhance the population of thin MoS 2 nanosheets ( Fig. 2a ). After this concentration step, 0.027 mg of MoS 2 flakes with thickness <5 nm remain, of which 24% are single-layer MoS 2 flakes as determined by AFM. This level of exfoliation is comparable to previous literature [32] and may be improved with the development of emerging techniques such as shear mixing [33] , [34] or ball milling [35] . After ultracentrifugation, dense iodixanol solution containing 2% w v −1 F68 was injected above the sedimented aggregates at the bottom of ultracentrifuge tube to separate and allow fractionation of the concentrated MoS 2 nanosheets. The extracted F68-MoS 2 dispersion was stable for several months. We also observed that when concentrated MoS 2 nanosheets were prepared using SC as the surfactant, there was no isolation of a SC-MoS 2 band ( Supplementary Fig. 2 ), which further illustrates the effectiveness of F68 as a dispersant for MoS 2 . 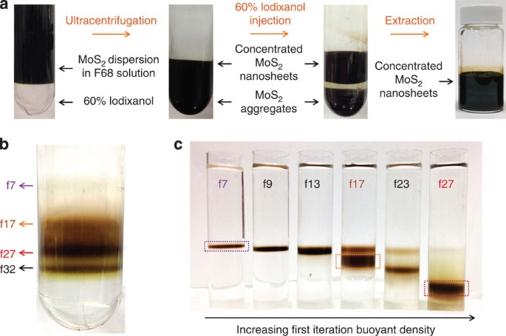Figure 2: Photographs of the experimental procedure. (a) Photographs of the concentration step for MoS2nanosheets. After ultrasonication, the MoS2dispersion is placed on top of 60% w v−1iodixanol as a step gradient and then ultracentrifuged at 32 kr.p.m. for 24 h. Subsequently, 60% w v−1iodixanol is injected to separate the concentrated MoS2nanosheets from the aggregates, and then extracted. The dispersion, gradient and injection solution all contain 2% w v−1F68. (b) Photograph of MoS2bands in an ultracentrifuge tube after the first iteration of density gradient ultracentrifugation (DGU). The concentrated MoS2solution was diluted by a factor of eight before ultracentrifugation to reveal the position of each band more clearly. (c) Photograph of the ultracentrifuge tubes after the second iteration of DGU. Fractions from the well-defined bands (f7, f17 and f27) and the relatively wider bands (f9, f13 and f23) from the first iteration are collected and used for the second iteration. The fractions from the dashed region are used for characterization. Figure 2: Photographs of the experimental procedure. ( a ) Photographs of the concentration step for MoS 2 nanosheets. After ultrasonication, the MoS 2 dispersion is placed on top of 60% w v −1 iodixanol as a step gradient and then ultracentrifuged at 32 kr.p.m. for 24 h. Subsequently, 60% w v −1 iodixanol is injected to separate the concentrated MoS 2 nanosheets from the aggregates, and then extracted. The dispersion, gradient and injection solution all contain 2% w v −1 F68. ( b ) Photograph of MoS 2 bands in an ultracentrifuge tube after the first iteration of density gradient ultracentrifugation (DGU). The concentrated MoS 2 solution was diluted by a factor of eight before ultracentrifugation to reveal the position of each band more clearly. ( c ) Photograph of the ultracentrifuge tubes after the second iteration of DGU. Fractions from the well-defined bands (f7, f17 and f27) and the relatively wider bands (f9, f13 and f23) from the first iteration are collected and used for the second iteration. The fractions from the dashed region are used for characterization. Full size image After the concentration step, the fractionated F68-MoS 2 solution was placed at the bottom of a linear density gradient and ultracentrifuged at 28 kr.p.m. for 12 h. The first iteration of DGU induces the F68-MoS 2 nanosheets to separate into multiple visible bands throughout the ultracentrifuge tube ( Fig. 2b ). These bands were recovered in 1 mm steps using a piston gradient fractionator and labelled with their position (that is, fractions were recovered starting from 6 mm above the first band and thus f7 indicates the fraction that encompasses the first band). For further refinement, three fractions from the most well-defined bands (f7, f17 and f27) and relatively wider bands (f9, f13 and f23) were extracted, and then placed at the top of a linear density gradient. The second iteration of DGU was performed at 41 kr.p.m. for 12 h, leading to the formation of well-defined MoS 2 bands at their corresponding isopycnic points (dashed regions in Fig. 2c ), which were then fractionated for characterization. The topmost band, which will later be shown to be highly enriched in single-layer MoS 2 , possesses a mass of 0.002 mg, which implies that DGU captures 30.8% of the exfoliated single-layer MoS 2 flakes (See Supplementary Discussion for more details on the calculation of the DGU yield). It should be noted that similar DGU results were achieved for other TMDs (for example, DGU of WS 2 , MoSe 2 and WSe 2 are shown in Supplementary Figs 3 and 4 ), thus demonstrating the generality of the copolymer-assisted DGU for thickness sorting of two-dimensional nanomaterials. Structure analysis of sorted MoS2 nanosheets High-angle annular dark field scanning transmission electron microscopy (HAADF-STEM) was used to verify the 2H structural phase and characterize atomic-level defects of the MoS 2 nanosheets. 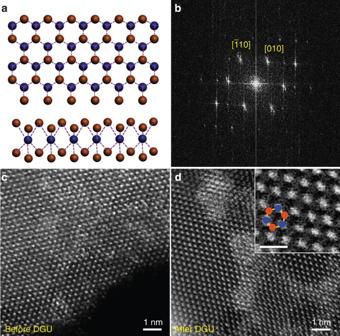Figure 3: Atomic structure of MoS2before and after DGU. (a) Schematic illustration of the 2H semiconducting crystal structure of MoS2shown from out-of-plane and perspective view (blue: Mo, brown: S). (b) Fast Fourier Transform of the STEM images. (c,d) HAADF-STEM images of MoS2flakes before and after DGU, respectively. The inset image shows the magnified STEM image after DGU. The blue and brown spheres indicate the position of Mo and S atoms, respectively (scale bar, 0.5 nm). Figure 3a shows a schematic illustration of the 2H structural phase with trigonal prismatic coordination. A Fast Fourier Transform from the HAADF-STEM image with two direction index is shown in Fig. 3b . Figure 3c,d show high resolution HAADF-STEM images of MoS 2 nanosheets before and after DGU. The inset in Fig. 3d shows the magnified STEM image with the position of Mo (blue) and S (brown) atoms. These STEM images reveal that the pristine 2H semiconducting structure of MoS 2 is preserved with minimal surface or edge defects following DGU processing [36] . Figure 3: Atomic structure of MoS 2 before and after DGU. ( a ) Schematic illustration of the 2H semiconducting crystal structure of MoS 2 shown from out-of-plane and perspective view (blue: Mo, brown: S). ( b ) Fast Fourier Transform of the STEM images. ( c , d ) HAADF-STEM images of MoS 2 flakes before and after DGU, respectively. The inset image shows the magnified STEM image after DGU. The blue and brown spheres indicate the position of Mo and S atoms, respectively (scale bar, 0.5 nm). Full size image Atomic force microscopy (AFM) was used to characterize the thickness and size of the sorted MoS 2 nanosheets. AFM images ( Fig. 4a ) indicate that the most buoyant fraction (f7) contains predominantly monolayers, while the less buoyant fraction (f17) primarily consists of MoS 2 multilayers. From the line profile, a monolayer MoS 2 flake in f7 has ~1 nm thickness. This measured thickness is slightly larger than previously reported values [2] , [4] , which is reasonable due to the presence of residual F68. 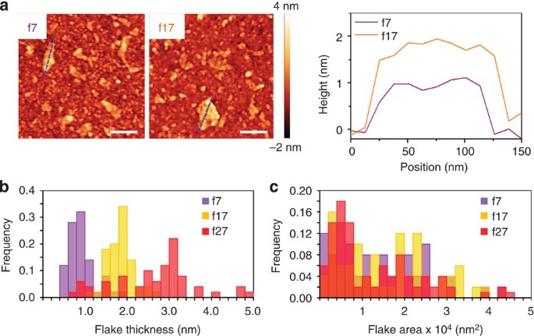Figure 4: Characterization of thickness and area distribution. (a) Atomic force microscopy (AFM) images of MoS2nanosheets from f7 (purple) and f17 (orange) on a SiO2substrate and the corresponding height profiles along the dashed lines (scale bar, 100 nm). (b) Flake thickness and (c) flake area histograms for f7 (purple), f17 (orange) and f27 (red) fractions obtained from the AFM images. Figure 4b,c show the AFM-measured thickness and area histograms for MoS 2 nanosheets from the f7, f17 and f27 fractions. These histograms were obtained from >100 individual MoS 2 flakes from each fraction. The average flake thicknesses for fractions f7, f17 and f27 are 1.02, 1.84 and 2.52 nm, respectively, thus demonstrating effective thickness sorting by DGU. In contrast, the flake area histograms show significant overlap, which is consistent with the buoyant density of two-dimensional nanomaterials being independent of lateral area (to corroborate the AFM lateral size histograms, scanning electron microscopy analysis was also performed; see Supplementary Fig. 9 ). Overall, it is evident that the MoS 2 DGU separation is driven by thickness instead of the lateral size with ~86% of the MoS 2 nanosheets from f7 having a thickness <1.2 nm, which corresponds to single layers of MoS 2 . Figure 4: Characterization of thickness and area distribution. ( a ) Atomic force microscopy (AFM) images of MoS 2 nanosheets from f7 (purple) and f17 (orange) on a SiO 2 substrate and the corresponding height profiles along the dashed lines (scale bar, 100 nm). ( b ) Flake thickness and ( c ) flake area histograms for f7 (purple), f17 (orange) and f27 (red) fractions obtained from the AFM images. Full size image On the basis of the measured thickness and buoyant density values, the MoS 2 experimental data are plotted with the geometrical buoyant density model in Fig. 5a . The experimental values (purple squares) imply a Pluronic F68 packing density σ of 0.244 nm −2 . Since the PPO chain of Pluronic F68 occupies an area of ~1.74 nm 2 on the MoS 2 surface, this packing density corresponds to ~42.5% surface coverage of Pluronic F68 (ref. 37 ). In Supplementary Table 2 , the surface coverage of F68 for WS 2 , MoSe 2 and WSe 2 are determined to be 61.4, 68.2 and 57.0%, respectively. These experimentally determined surface coverages correlate with the relative hydrophobicity of each TMD. In particular, the most hydrophilic MoS 2 surface shows the lowest F68 surface coverage, which is consistent with expectations since F68 interacts with the TMD surface via its hydrophobic PPO chains. 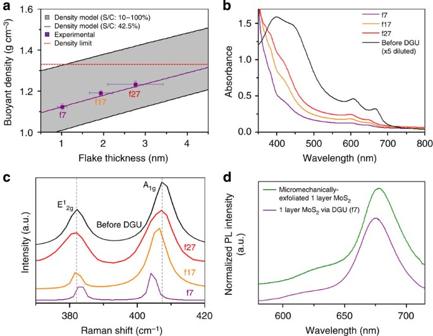Figure 5: Buoyant density analysis and optical properties. (a) Experimental data (purple squares) are plotted with the buoyant density model using a surface coverage variation from 10–100% (black lines). The surface coverage of F68 on the MoS2surface determined from the experimental data, which corresponds to ~42.5%, is also shown as a purple line. (b) Optical absorbance spectra of fractions f7 (purple), f17 (orange) and f27 (red), and the MoS2dispersion before separation (black). (c) Raman spectra of each fraction showing the shifts in the in-plane and out-of-plane vibrational modes as a function of MoS2thickness. (d) Photoluminescence spectra of fraction f7 (purple) compared with a micromechanically exfoliated monolayer MoS2(green). Figure 5: Buoyant density analysis and optical properties. ( a ) Experimental data (purple squares) are plotted with the buoyant density model using a surface coverage variation from 10–100% (black lines). The surface coverage of F68 on the MoS 2 surface determined from the experimental data, which corresponds to ~42.5%, is also shown as a purple line. ( b ) Optical absorbance spectra of fractions f7 (purple), f17 (orange) and f27 (red), and the MoS 2 dispersion before separation (black). ( c ) Raman spectra of each fraction showing the shifts in the in-plane and out-of-plane vibrational modes as a function of MoS 2 thickness. ( d ) Photoluminescence spectra of fraction f7 (purple) compared with a micromechanically exfoliated monolayer MoS 2 (green). Full size image Spectroscopic characterization Following DGU, optical absorbance spectra for fractions f7, f17 and f27 in addition to the MoS 2 dispersion before separation were measured ( Fig. 5b ). The direct MoS 2 excitonic transition peaks at ~610 and ~660 nm are present in all of the samples after DGU, further confirming that the original 2H-MoS 2 crystal structure was maintained through the separation process. The two absorption peaks between 600 and 700 nm are attributed to the excitonic peaks of MoS 2 . The weaker optical intensity of these peaks from f7, f17 and f27 are due to the relatively small concentration of MoS 2 in the solution following DGU. In addition, the blue shift observed in these peaks is consistent with the smaller lateral flake size following DGU (See Supplementary Fig. 9 ) [38] , [39] , [40] , [41] , and the strong absorption <400 nm is attributed to the density gradient medium (that is, iodixanol). Each MoS 2 fraction was also characterized by Raman spectroscopy ( Fig. 5c ). In this case, MoS 2 films were prepared by vacuum filtration and transferred onto a SiO 2 substrate, at which point Raman spectra were obtained using a beam size of ~1 μm and an excitation wavelength of 514 nm. The Raman spectra from the unsorted MoS 2 sample and fraction f27 show two peaks, specifically the in-plane E 1 2 g mode at ~382 cm −1 and the out-of-plane A 1 g mode at ~407 cm −1 , which are comparable to those of bulk MoS 2 (ref. 16 ). As the number of layers decreases, the E 1 2 g mode is stiffened and the A 1 g mode is softened, such that the peaks from fraction f7 are shifted to ~384 cm −1 and ~404 cm −1 , respectively [16] . In addition, the width of these two peaks is reduced in the more buoyant fractions, which confirms that the flake thickness homogeneity is improved by DGU. To further verify the isolation of MoS 2 monolayers, photoluminescence spectroscopy was performed on fraction f7 (purple line) using an excitation wavelength of 514 nm ( Fig. 5d ). For comparison, a photoluminescence spectrum was obtained under identical measurement conditions from a micromechanically exfoliated monolayer of MoS 2 (green line), and both spectra were normalized using their Raman spectra (optical microscopy image of the micromechanically exfoliated monolayer MoS 2 is shown in Supplementary Fig. 6 ). The photoluminescence spectra from each fraction show two peaks with comparable intensities at ~610 and ~660 nm that are well correlated with the MoS 2 excitonic transitions. WS 2 nanosheets were similarly characterized following DGU, where photoluminescence was also observed from the most buoyant fractions (See Supplementary Fig. 7 ). In conclusion, isopycnic DGU enables solution-phase preparation of controlled thickness TMDs. Specifically, the amphiphilic block copolymer Pluronic F68 increases the hydration and thus reduces the effective buoyant density of TMDs into the range of standard density gradient media. Thickness sorting of TMDs is confirmed with AFM and Raman spectroscopy, resulting in the emergence of photoluminescence from the most buoyant single-layered nanosheets. Furthermore, atomic-resolution STEM imaging verifies that the resulting thickness-sorted TMDs possess high crystal quality with low surface and edge defect density. Since DGU has proven industrial scalability, this approach holds promise for the solution-phase production of monolayered TMDs in emerging large-volume applications including photovoltaics, catalysis, biotechnology and electronics. Dispersion and density gradient ultracentrifugation One gram of MoS 2 powder (American Elements) was dispersed in 70 ml of 2% w v −1 Pluronic F68 (BASF) aqueous solution via ultrasonication using a 0.125-inch tip in a steel beaker at 25 W for 2 h. Then, 32 ml of dispersion was carefully added on top of a 6 ml underlayer of 60% w v −1 iodixanol and ultracentrifuged at 32 kr.p.m. for 24 h at 22 °C using a SW32 Ti rotor (Beckman-Coulter). Following ultracentrifugation, 3 ml of 60% w v −1 iodixanol was injected to separate ~10 ml of concentrated MoS 2 nanosheet solution, which was then fractionated using a piston gradient fractionator (BioComp Instruments). For the first iteration, the concentrated MoS 2 solution was diluted to contain 46% w v −1 iodixanol, and placed under a linear density gradient of 25–45% w v −1 iodixanol. The linear density gradient was then ultracentrifuged at 28 kr.p.m. for 12 h at 22 °C. Following the first iteration, each fraction was diluted to contain 9% w v −1 iodixanol and placed on top of a linear density gradient of 30–50% w v −1 iodixanol for the second iteration. The linear density gradient was then ultracentrifuged in an SW41 Ti rotor (Beckman-Coulter) at 41 kr.p.m. for 12 h. All density gradient and injection solutions contained 2% w v −1 F68. Sample preparation for scanning transmission electron microscopy MoS 2 dispersions from each step (after sonication before DGU and after DGU) were collected and placed in 20 k MWCO dialysis cassettes (Thermo Scientific) and dialysed in 750 ml of 2% w v −1 F68 aqueous bath for 24 h to remove the density gradient medium. To remove the surfactant, MoS 2 dispersions were mixed with isopropyl alcohol for 24 h, filtered through mixed cellulose ester membranes (Millipore, 50 nm pore size), and rinsed with deionized water. The resulting aggregated MoS 2 nanosheets were then bath sonicated (Branson ultrasonic cleaner 3510) to redisperse in deionized water. Sample preparation for atomic force microscopy The separated MoS 2 fractions were dialysed in 750 ml of 2% w v −1 SC bath for 48 h to enable surfactant exchange. Before deposition, a SiO 2 substrate was rinsed with acetone, methanol and deionized water and immersed in 2% polyethylenimine for 2 min to form a self-assembled monolayer. The substrate was then dried under nitrogen gas, rinsed in deionized water and dried again. The samples were drop casted onto polyethylenimine-treated SiO 2 substrate for 5 min, dried under nitrogen gas, rinsed in deionized water, dried again and annealed at 250 °C for 1 h to remove residual surfactants and iodixanol. To increase the areal density of MoS 2 flakes, this process was repeated 5–10 times. Sample preparation for Raman and photoluminescence spectroscopy MoS 2 films were prepared via the vacuum filtration method. In particular, 2 ml of MoS 2 dispersion was filtered. The residual surfactant and iodixanol were then removed by rinsing with 30 ml of deionized water. The resulting film was immersed in ethanol and pressed firmly onto a SiO 2 substrate for 10 min by applying pressure with a 1.5 kg weight. To remove the membrane, the substrate was suspended above a boiling acetone bath at 85 °C at a 45° angle. After 15 min, the substrate was rinsed with ethanol, acetone, ethanol again and deionized water, and then dried with nitrogen gas. How to cite this article: Kang, J. et al. Thickness sorting of two-dimensional transition metal dichalcogenides via copolymer-assisted density gradient ultracentrifugation. Nat. Commun. 5:5478 doi: 10.1038/ncomms6478 (2014).